PINK1 deficiency sustains cell proliferation by reprogramming glucose metabolism through HIF1 PTEN-induced kinase-1 (PINK1) is a Ser/Thr kinase implicated in familial early-onset Parkinson’s disease, and was first reported as a growth suppressor. PINK1 loss-of-function compromises both mitochondrial autophagy and oxidative phosphorylation. Here we report that PINK1 deficiency triggers hypoxia-inducible factor-1α (HIF1α) stabilization in cultured Pink1 −/− mouse embryonic fibroblasts and primary cortical neurons as well as in vivo . This effect, mediated by mitochondrial reactive oxygen species, led to the upregulation of the HIF1 target, pyruvate dehydrogenase kinase-1, which inhibits PDH activity. Furthermore, we show that HIF1α stimulates glycolysis in the absence of Pink1 , and that the promotion of intracellular glucose metabolism by HIF1α stabilization is required for cell proliferation in Pink1 −/− mice. We propose that loss of Pink1 reprograms glucose metabolism through HIF1α, sustaining increased cell proliferation. Parkinson’s disease (PD) is the second most common neurodegenerative disease, affecting 1–2% of people over 65 years of age. PD is characterized by the loss of dopaminergic neurons and the development of intracellular aggregates of the protein α-synuclein. Currently, it is widely accepted that mitochondrial dysfunction is a key factor in PD pathogenesis [1] . While the vast majority of PD cases are sporadic, 5–10% of cases are inherited through mutations in PD-related genes. There is now compelling evidence supporting the notion that the autosomal recessive early-onset PD-related genes PTEN-induced kinase-1 ( PINK1 ) and PARKIN are key regulators of the mitochondrial quality control [2] , [3] . Full-length PINK1 localizes to the mitochondrial outer membrane [3] , [4] , where it interacts—in a phosphorylation-dependent manner—with PARKIN [5] , [6] , both acting on the same pathway as a quality control system to preserve mitochondrial integrity on mitochondrial membrane potential (Δψ m ) collapse. Thus, loss of PINK1, or disease-relevant mutations in PINK1 gene, compromises mitochondrial autophagy [7] , [8] , [9] , [10] , as well as mitochondrial oxidative phosphorylation, predominantly at the level of complex I [11] , [12] . Besides its role in PD, PINK1 was reported to have a growth suppressive function [13] through a yet unravelled mechanism. Given that cell proliferation requires, among other metabolic adaptations, a high glycolytic rate [14] and, in view of its mitochondrial protection role, we hypothesized that PINK1 might act by modulating glycolysis. Here, we show that the loss of Pink1 reprograms glucose metabolism through hypoxia-inducible factor-1α (HIF1α) to stimulate glycolysis. Unexpectedly, we found that the glycolytic reprogramming is required for the increased cell proliferation observed on loss of Pink1 . Loss of Pink1 stimulates glucose metabolism To elucidate whether PINK1 regulates glucose metabolism, we first obtained Pink1 −/− ( Pink1 knockout or KO) and Pink1 +/+ (wild type or WT) primary mouse embryonic fibroblasts (MEF) from the same offspring. The rates of glucose uptake ( Fig. 1a ) and glycolysis ( Fig. 1b,c ) in Pink1 KO MEF were approximately twofold higher when compared with WT. Instead, the rate of glucose utilization through the pentose–phosphate pathway (PPP) was ~45% lower in Pink1 KO MEF than in WT ( Fig. 1d ), indicating the shift of glucose-6-phosphate consumption from PPP towards glycolysis that also takes place in other biological settings [15] . To extend these findings to non-proliferating cells, we next assessed glucose metabolism in cultured primary cortical neurons. As shown in Fig. 1e–g , loss of Pink1 in neurons triggered a ~twofold increase in the rates of glucose uptake and glycolysis when compared with WT. The flux of glucose consumption through the PPP was reduced in a similar extent in Pink1 KO neurons ( Fig. 1h ), suggesting metabolic shift from PPP to glycolysis in neurons. We next sought to confirm the enhanced glucose metabolism in vivo . We found that Pink1 KO mice were slightly hypoglycaemic ( Fig. 1i ) and hyperlactatemic ( Fig. 1j ). In addition, the rate of 14 C-lactate appearance in the blood from acutely injected [U- 14 C]glucose mice was higher in Pink1 KO than in WT ( Fig. 1k ). Together, these results indicate that the loss of Pink1 causes a metabolic reprogramming that promotes glucose uptake and glycolysis. 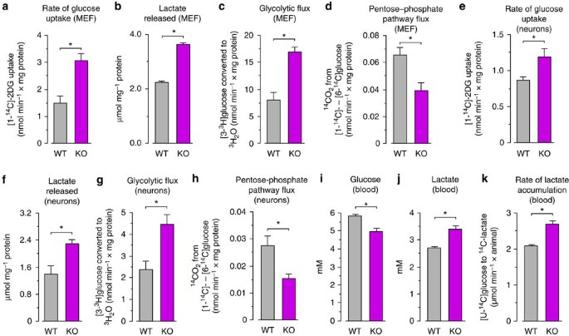Figure 1: Enhanced glucose metabolism on loss ofPink1. The rate of glucose uptake (a,e), lactate released after 4 h of incubation (b,f), glycolytic flux (c,g) and pentose–phosphate flux (d,h) were assessed in MEF and mouse cortical neurons in primary culture, as indicated, obtained from either WT orPink1KO (Pink1−/−) mice. Blood concentrations of glucose (i) and lactate (j), and the rate of14C-lactate appearance in the blood from acutely injected [U-14C]glucose in the tail vein (k) of WT andPink1KO mice were analysed. Data are expressed as mean±s.e.m. *P<0.05 (Student’st-test;n=3–4 independent experiments). Figure 1: Enhanced glucose metabolism on loss of Pink1 . The rate of glucose uptake ( a , e ), lactate released after 4 h of incubation ( b , f ), glycolytic flux ( c , g ) and pentose–phosphate flux ( d , h ) were assessed in MEF and mouse cortical neurons in primary culture, as indicated, obtained from either WT or Pink1 KO ( Pink1 −/− ) mice. Blood concentrations of glucose ( i ) and lactate ( j ), and the rate of 14 C-lactate appearance in the blood from acutely injected [U- 14 C]glucose in the tail vein ( k ) of WT and Pink1 KO mice were analysed. Data are expressed as mean±s.e.m. * P <0.05 (Student’s t -test; n =3–4 independent experiments). Full size image Glucose-utilizing enzymes and HIF1α are altered on loss of Pink1 To investigate whether the changes in glucose metabolism observed by the loss of Pink1 were associated with alterations in the expression of glycolytic enzymes, we next analysed the relative messenger RNA (mRNA) abundance of key glucose-metabolizing enzymes. As shown in Fig. 2a , glucose transporter-1 ( Glut1 ), glucose transporter-3 ( Glut3 ), hexokinase-2 ( Hk2 ) and glyceraldehyde-3-phosphate dehydrogenase ( Gapdh ) mRNA abundances, relative to those of the housekeeping ß-Actin , were ~1.5–2.5-fold higher in Pink1 KO MEF when compared with WT. The relative mRNA abundance of other key glycolytic enzymes, including 6-phosphofructo-2-kinase/fructose-2,6-bisphosphatase-3, enolase-1 and lactate dehydrogenase-a, but not that of hexokinase-1), albeit very slightly, were also higher in the Pink1 KO MEF than in WT ( Supplementary Fig. 1a ). The protein levels of GLUT1, HK2 and GAPDH were also increased in the Pink1 KO MEF ( Fig. 2b ; Supplementary Fig. 1b ); GLUT3 protein was undetectable in MEF (not shown). As these transporters and enzymes are well-known targets of hypoxia-inducible factor-1 (HIF1), we next investigated the abundance of its α-subunit (HIF1α) that is amenable to regulation by protein stability [16] . As shown in Fig. 2b , HIF1α protein was increased in MEF lacking Pink1 (see, also, Supplementary Fig. 1b ). Since this effect cannot be ascribed to a putative increase in Hif1 α mRNA abundance ( Hif1 α levels in Pink1 KO MEF were found to be 0.49 plus or minus (±) 0.07-fold, normalized to ß-actin , when compared with WT; n =3), our data indicate the stabilization of HIF1α in the Pink1 KO MEF. Likewise, cultured primary neurons from the Pink1 KO mice had ~1.4–1.8-fold enhancement in the mRNA abundances of Glut1 , Glut3 , Hk2 and Gapdh when compared with WT ( Fig. 2c ). The corresponding proteins were increased accordingly ( Fig. 2d ; Supplementary Fig. 1c ). In Pink1 KO neurons, HIF1α protein—but not its mRNA ( Hif α levels in Pink1 KO neurons were found to be 0.43±0.11-fold, normalized to ß-actin , when compared with WT; n =3)—was higher than in WT ( Fig. 2d ; Supplementary Fig. 1c ). To extend our observations to in vivo settings, we confirmed the upregulation of GLUT1, GLUT3 and HIF1α in skeletal muscle of Pink1 KO mice ( Figs 1d , 2e ). In addition, we performed a microRNA (miR) transcription profiling in Pink1 KO mice brain, which revealed significantly elevated several miRs, such as miR-30b-5p , miR-26b-5p , miR-27a-3p , miR-181c-5p , miR-494-3p and miR-30d-5p that are reported to modulate HIF1α repression [17] ( Supplementary Table 1 ). Thus, our data indicate HIF1α stabilization in the Pink -null mice, and HIF1α-target proteins enhancement likely contributing to the observed glucose metabolism reprogramming. 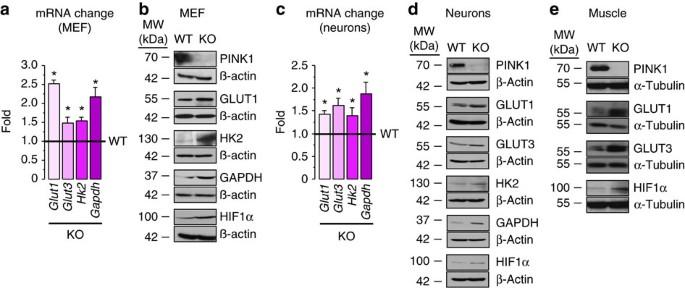Figure 2: Glucose-utilizing enzymes and HIF1α are altered byPink1loss. Quantitative real-time PCR (RT–qPCR analysis of the relative mRNA abundances ofGlut1,Glut3,Hk2andGapdhin WT andPink1KO mice MEF (a) or neurons (c).ß-ActinmRNA was used for normalization, and thePink1KO data are expressed as the change relative to WT. Western blot analysis of the protein abundances of PINK1, GLUT1, GLUT3 (not detectable in MEF), HK2, GAPDH and HIF1α in WT andPink1-nullmice MEF (b) or neurons (d); ß-Actin was used as loading control. (e) Western blot against PINK1, GLUT1, GLUT3 and HIF1α in WT andPink1KO mice skeletal muscle samples; α-Tubulin was used as loading control. Only representative western blots are shown per condition; the replicates and the semi-quantitative estimation of the band intensities are shown in theSupplementary Information. The mean±s.e.m. values of the mRNA data were calculated from the fold change of eachß-Actin-normalized transcript abundance in thePink1KO samples versus that in the WT. Thus, in all cases, the WT values were considered=1.00. *P<0.05 versus the corresponding WT (Student’st-test;n=3–4 independent experiments). Figure 2: Glucose-utilizing enzymes and HIF1α are altered by Pink1 loss. Quantitative real-time PCR (RT–qPCR analysis of the relative mRNA abundances of Glut1 , Glut3 , Hk2 and Gapdh in WT and Pink1 KO mice MEF ( a ) or neurons ( c ). ß-Actin mRNA was used for normalization, and the Pink1 KO data are expressed as the change relative to WT. Western blot analysis of the protein abundances of PINK1, GLUT1, GLUT3 (not detectable in MEF), HK2, GAPDH and HIF1α in WT and Pink1-null mice MEF ( b ) or neurons ( d ); ß-Actin was used as loading control. ( e ) Western blot against PINK1, GLUT1, GLUT3 and HIF1α in WT and Pink1 KO mice skeletal muscle samples; α-Tubulin was used as loading control. Only representative western blots are shown per condition; the replicates and the semi-quantitative estimation of the band intensities are shown in the Supplementary Information . The mean±s.e.m. values of the mRNA data were calculated from the fold change of each ß-Actin -normalized transcript abundance in the Pink1 KO samples versus that in the WT. Thus, in all cases, the WT values were considered=1.00. * P <0.05 versus the corresponding WT (Student’s t -test; n =3–4 independent experiments). Full size image HIF1α is required for increased glycolysis on Pink1 loss To directly demonstrate the involvement of HIF1α in the glycolytic phenotype caused by loss of Pink1 , we explored the consequences of its removal by RNA interference . As shown in Fig. 3a , transfection of MEF with a small interfering RNA (siRNA) against Hif α ( siHif1 α) showed an ~60% decrease in Hif1 α mRNA abundance when compared with controls. This effect was selective since siHif1 α was unable to knockdown the HIF1α protein that was expressed from a mutant form of Hif1 α cDNA harbouring silent mutations on its siRNA-target region ( Fig. 3b ; Supplementary Fig. 2a ). HIF1α knockdown fully prevented the increase in the Glut1 , Glut3 , Hk2 and Gapdh mRNA abundance ( Fig. 3c ), and in the GLUT1 and GAPDH ( Fig. 3d ; Supplementary Fig. 2b ) protein abundance of the Pink1 KO MEF. Furthermore, the increased lactate released ( Fig. 3e ) and glycolytic rate ( Fig. 3f ) promoted by PINK1 loss-of-function was rescued by knocking down HIF1α. Likewise, knocking down HIF1α in primary neurons ( Fig. 3g ; Supplementary Fig. 2c ) fully abolished the increase in the glycolytic rate exerted by PINK loss-of-function ( Fig. 3h ). Together, these data strongly suggest that HIF1α is required for the enhanced glycolytic phenotype caused by the loss of Pink1 . 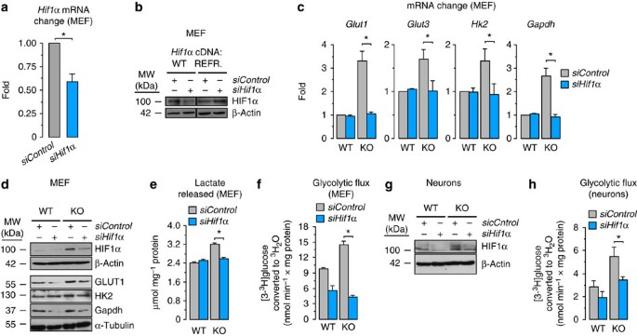Figure 3: HIF1α is required for increased glycolysis byPink1loss. AnsiHif1α was used to evaluate its involvement in the glycolytic phenotype ofPink1KO cells. (a) RT–qPCR analysis ofHif1α mRNA abundance in MEF transfected withsiHif1α, orsiControl(100 nM), after 72 h. (b)siHif1α effectively knockdowns expressedHif1α cDNA WT, but not aHif1α cDNA silent mutant form refractory tosiHif1α (Hif1α cDNA REFR.) in mice MEF. (c) RT–qPCR analysis of the relative mRNA abundances ofGlut1,Glut3,Hk2andGapdhin WT andPink1KO mice MEF transfected withsiControlorsiHif1α.ß-ActinmRNA was used for normalization, and all data are expressed as the change relative to WT-siControl. (d) Western blot against HIF1α in WT and inPink1KO mice MEF transfected withsiHif1α orsiControlshows the efficacy of thesiHif1α at knocking down endogenous HIF1α; ß-actin was used as loading control. As shown,siHif1α partially prevented the increase in GLUT1, HK2 and GAPDH protein abundances. The increased rate of lactate released after 4 h of incubation (e) and glycolytic flux (f) observed in thePink1KO MEF was prevented bysiHif1α.siHif1α was also effective at preventing the endogenous increased HIF1α protein (g), as well as the increased glycolytic flux (h) observed inPink1KO primary neurons. Only representative western blots are shown; the replicates and the semi-quantitative estimation of the band intensities are shown in theSupplementary Information. The mean±s.e.m. values of the mRNA data were calculated from the fold change of eachß-actin-normalized transcript abundance in thePink1KO samples versus that in the WT (a) or WT-siControl(c); thus, in all these cases, the WT (a) or WT-siControl(c) values were considered=1.00. Only the statistical analysis results of thesiHif1α versussiControl(in KO) values (mean±s.e.m.) are shown inc,e,f,h, since the comparison KO versus WT under control conditions was previously shown inFig. 2a,Fig. 1b,c,g, respectively. *P<0.05 (Student’st-test;n=3–4 independent experiments). Figure 3: HIF1α is required for increased glycolysis by Pink1 loss. An siHif1 α was used to evaluate its involvement in the glycolytic phenotype of Pink1 KO cells. ( a ) RT–qPCR analysis of Hif1 α mRNA abundance in MEF transfected with siHif1 α, or siControl (100 nM), after 72 h. ( b ) siHif1 α effectively knockdowns expressed Hif1 α cDNA WT, but not a Hif1 α cDNA silent mutant form refractory to siHif1 α ( Hif1 α cDNA REFR.) in mice MEF. ( c ) RT–qPCR analysis of the relative mRNA abundances of Glut1 , Glut3 , Hk2 and Gapdh in WT and Pink1 KO mice MEF transfected with siControl or siHif1 α. ß-Actin mRNA was used for normalization, and all data are expressed as the change relative to WT- siControl . ( d ) Western blot against HIF1α in WT and in Pink1 KO mice MEF transfected with siHif1 α or siControl shows the efficacy of the siHif1 α at knocking down endogenous HIF1α; ß-actin was used as loading control. As shown, siHif1 α partially prevented the increase in GLUT1, HK2 and GAPDH protein abundances. The increased rate of lactate released after 4 h of incubation ( e ) and glycolytic flux ( f ) observed in the Pink1 KO MEF was prevented by siHif1 α. siHif1 α was also effective at preventing the endogenous increased HIF1α protein ( g ), as well as the increased glycolytic flux ( h ) observed in Pink1 KO primary neurons. Only representative western blots are shown; the replicates and the semi-quantitative estimation of the band intensities are shown in the Supplementary Information . The mean±s.e.m. values of the mRNA data were calculated from the fold change of each ß-actin -normalized transcript abundance in the Pink1 KO samples versus that in the WT ( a ) or WT- siControl ( c ); thus, in all these cases, the WT ( a ) or WT- siControl ( c ) values were considered=1.00. Only the statistical analysis results of the siHif1 α versus siControl (in KO) values (mean±s.e.m.) are shown in c , e , f , h , since the comparison KO versus WT under control conditions was previously shown in Fig. 2a , Fig. 1b,c,g , respectively. * P <0.05 (Student’s t -test; n =3–4 independent experiments). Full size image Mitochondrial ROS mediate HIF1α stabilization on Pink1 loss To understand how the lack of PINK1 upregulated HIF1α, we first confirmed the defects in both mitochondrial respiratory chain ( Fig. 4a ) and inner membrane potential ( Fig. 4b ) of Pink1 KO MEF that were previously reported in similar settings [11] , [18] . Moreover, we found that pyruvate dehydrogenase kinase-1 (PDK1) protein abundance, a known HIF1-target [19] , was higher in Pink1 KO MEF when compared with WT ( Fig. 4c ; Supplementary Fig. 2e ). In addition, we found that the increase in PDK1 protein was abolished by knocking down HIF1α ( Fig. 4c ; Supplementary Fig. 2e ). Since PDK1 phosphorylates PDH, complex inhibiting its activity, we next determined PDH activity in the Pink1 KO MEF. As shown in Fig. 4d , PDH activity was ~80% lower in Pink1 KO cells when compared with WT, and this effect was ablated by HIF1α knockdown. Thus, through HIF1, PINK1 deficiency inhibits PDH activity, which likely contributes to a positive loop of mitochondrial impairment. Confirming previous work [18] , we found that the rates of H 2 O 2 and mitochondrial O 2 ·– detected were higher in MEF from Pink1 KO mice than in the WT ( Fig. 4e,f ). Since these reactive oxygen species (ROS) stabilize HIF1α [20] , [21] , [22] , we sought to assess whether mitochondrial ROS mediated the enhancement of HIF1α observed by the loss of PINK1. As shown in Fig. 4g , mitochondrial O 2 ·– detection was reduced either by incubating MEF with a plasma membrane permeable form of glutathione (glutathione ethyl ester, GSH-EE), or by expressing mitochondrial-tagged forms of glutamate–cysteine ligase ( mitoGCL ) [23] or catalase ( mitoCAT ). As depicted in Fig. 4h and Supplementary Fig. 2f , the increase in HIF1α protein observed in Pink1 KO MEF was decreased not only by the whole-cell ROS scavenger GSH-EE, but also by selectively removing ROS in mitochondria with mitoGCL or mitoCAT . Thus, mitochondrial-derived ROS accounts for HIF1α protein stabilization caused by Pink1 loss. 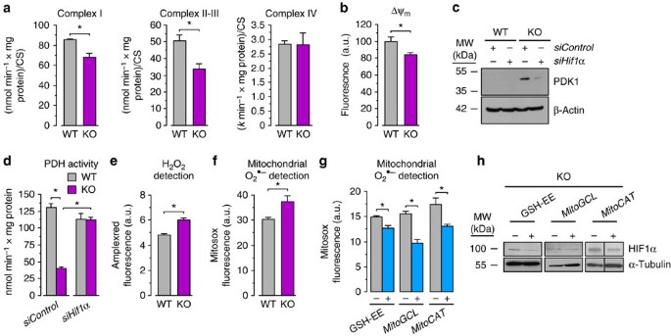Figure 4: Mitochondrial ROS mediate HIF1α stabilization byPink1loss. (a) Mitochondrial respiratory chain complexes activity values normalized to citrate synthase (CS), and (b) mitochondrial inner membrane potential (Δψm) in WT andPink1KO mice MEF. (c) Western blot against PDK1 and HIF1α in WT andPink1KO MEF transfected withsiHif1α (or itssiControl); ß-actin was used as loading control. (d) PDH complex activity in WT andPink1KO MEF transfected withsiHif1α orsiControl. Rate of whole-cell H2O2(e) and mitochondrial O2·−(f) detection in WT andPink1KO MEF. (g) Detection of mitochondrial O2·−using the mitochondrial-specific probe MitoSox in MEF incubated in the absence (−) or in the presence (+) of the plasma membrane permeable GSH-EE, or by expressing mitochondrial-tagged forms of glutamate-cysteine ligase, (+mitoGCL; empty vector, pIRES2–EGFP, denoted as −) or catalase (+mitoCAT; empty vector denoted as −), shows effective mitochondrial ROS removal. (h) Western blot against HIF1α inPink1KO MEF incubated with (or without) GSH-EE, or transfected with empty vector,mitoGCLormitoCAT, showing reduction in HIF1α protein abundance by the treatments that remove mitochondrial ROS; α-TUBULIN was used as loading control. Only representative western blots are shown; the replicates and the semi-quantitative estimation of the band intensities are shown in theSupplementary Information. Data are expressed as mean±s.e.m. *P<0.05 (Student’st-test;n=3–4 independent experiments). Figure 4: Mitochondrial ROS mediate HIF1α stabilization by Pink1 loss. ( a ) Mitochondrial respiratory chain complexes activity values normalized to citrate synthase (CS), and ( b ) mitochondrial inner membrane potential (Δψ m ) in WT and Pink1 KO mice MEF. ( c ) Western blot against PDK1 and HIF1α in WT and Pink1 KO MEF transfected with siHif1 α (or its siControl ); ß-actin was used as loading control. ( d ) PDH complex activity in WT and Pink1 KO MEF transfected with siHif1 α or siControl . Rate of whole-cell H 2 O 2 ( e ) and mitochondrial O 2 ·− ( f ) detection in WT and Pink1 KO MEF. ( g ) Detection of mitochondrial O 2 ·− using the mitochondrial-specific probe MitoSox in MEF incubated in the absence (−) or in the presence (+) of the plasma membrane permeable GSH-EE, or by expressing mitochondrial-tagged forms of glutamate-cysteine ligase, (+ mitoGCL ; empty vector, pIRES2–EGFP, denoted as −) or catalase (+ mitoCAT ; empty vector denoted as −), shows effective mitochondrial ROS removal. ( h ) Western blot against HIF1α in Pink1 KO MEF incubated with (or without) GSH-EE, or transfected with empty vector, mitoGCL or mitoCAT , showing reduction in HIF1α protein abundance by the treatments that remove mitochondrial ROS; α-TUBULIN was used as loading control. Only representative western blots are shown; the replicates and the semi-quantitative estimation of the band intensities are shown in the Supplementary Information . Data are expressed as mean±s.e.m. * P <0.05 (Student’s t -test; n =3–4 independent experiments). Full size image Increased cell proliferation on loss of Pink1 requires HIF1α Given that PINK1 is a growth-suppressor protein [13] and that increased glucose utilization supports cell growth [14] through HIF1 (ref. 16) [16] , we next sought to determine whether the observed increased rate of glycolysis in Pink1 KO cells was associated with an increase in cell proliferation. To achieve this, we evaluated the rate of bromo-deoxy-uridine (BrdU) incorporation into DNA, the proportion of each cell cycle phase, and cell growth in Pink1 KO MEF in the absence or in the presence of the glucose-metabolizing inhibitor, 2-deoxyglucose (2DG). As depicted in Fig. 5a , Pink1 KO MEF showed a higher rate of BrdU incorporation, decreased G 0 /G 1 phase, increased S and G 2 /M phases and higher rate of proliferation ( Fig. 5b ) when compared with WT; moreover, 2DG fully abolished Pink1 KO-mediated increase in cell proliferation ( Fig. 5a,b ), indicating the requirement of glucose utilization for Pink1 KO-induced cell proliferation. In addition, the increased proliferation rate of the Pink1 KO MEF was prevented by knocking down HIF1α ( Fig. 5c,d ), indicating the requirement of HIF1α stabilization for Pink1 KO-induced cell proliferation. To confirm the high proliferative status in vivo , we analysed the neurogenic subventricular zone (SVZ) in the Pink1 KO mouse brain. As shown in Fig. 5e , we observed a ~twofold increase in Ki67-immunostained cells that were positive for the stem cell marker Sox2, confirming enhanced proliferation rate of neural stem cells in vivo by Pink1 loss. Thus, our data shows that the loss of PINK1 causes an increase in cell proliferation, for which both glucose utilization and HIF1α are required. Primary neurons, obtained from the Pink1 KO mice, showed higher mitochondrial-derived ROS than WT ( Fig. 6a ), likely contributing—such as in MEF—to HIF1α stabilization. However, in line with their post-mitotic status, these Pink1 KO neurons showed unaltered their rate of BrdU incorporation rate ( Fig. 6b ); we found, instead an increased apoptotic cell death rate ( Fig. 6c ). Thus, the metabolic re-wiring caused by PINK1 loss-of-function, being unable to support proliferation in post-mitotic neurons, would likely be involved in a death phenotype. 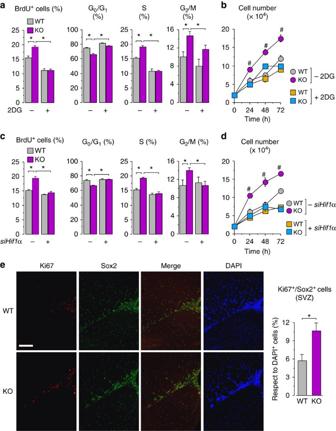Figure 5: Increased cell proliferation byPink1loss requires HIF1α. (a) Proportion of BrdU incorporation into DNA and cell cycle phases, and (b) cell growth in WT andPink1KO MEF after 72 h in the absence (denoted as -2DG) or in the presence (+2DG) of the glucose-metabolizing inhibitor, 2-deoxyglucose (2DG, 1 mM). (c) Proportions of BrdU incorporation into DNA and cell cycle phases, and (d) cell growth in WT andPink1KO MEF 72 h after transfection withsiHif1α (+siHif1α) orsiControl(denoted as -siHif1α). (e) Ki67, Sox2 and DAPI immunostaining in the subventricular zone of WT andPink1KO mouse brain, and the corresponding quantification. *P<0.05;#P<0.05 versus all other conditions (analysis of variance followed by Bonferroni test;n=3–4 independent experiments). All data are expressed as mean±s.e.m. Scale bar, 100 μm. Figure 5: Increased cell proliferation by Pink1 loss requires HIF1α. ( a ) Proportion of BrdU incorporation into DNA and cell cycle phases, and ( b ) cell growth in WT and Pink1 KO MEF after 72 h in the absence (denoted as -2DG) or in the presence (+2DG) of the glucose-metabolizing inhibitor, 2-deoxyglucose (2DG, 1 mM). ( c ) Proportions of BrdU incorporation into DNA and cell cycle phases, and ( d ) cell growth in WT and Pink1 KO MEF 72 h after transfection with siHif1 α (+ siHif1 α) or siControl (denoted as - siHif1 α). ( e ) Ki67, Sox2 and DAPI immunostaining in the subventricular zone of WT and Pink1 KO mouse brain, and the corresponding quantification. * P <0.05; # P <0.05 versus all other conditions (analysis of variance followed by Bonferroni test; n =3–4 independent experiments). All data are expressed as mean±s.e.m. Scale bar, 100 μm. 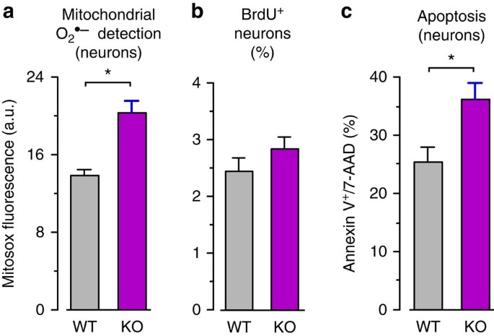Figure 6: Loss of Pink1 increases mitochondrial ROS and apoptosis in neurons. (a) Rate of mitochondrial O2·–detection in WT andPink1KO mice primary neurons. (b) Proportion of BrdU incorporation into DNA of WT andPink1KO neurons. (c) Proportion of apoptosis in WT andPink1KO neurons, as assessed by the proportion of annexin V-positive/7-AAD-negative cells, determined by flow cytometry. Data are expressed as mean±s.e.m. *P<0.05 (Student’st-test;n=3–4 independent experiments). Full size image Figure 6: Loss of Pink1 increases mitochondrial ROS and apoptosis in neurons. ( a ) Rate of mitochondrial O 2 ·– detection in WT and Pink1 KO mice primary neurons. ( b ) Proportion of BrdU incorporation into DNA of WT and Pink1 KO neurons. ( c ) Proportion of apoptosis in WT and Pink1 KO neurons, as assessed by the proportion of annexin V-positive/7-AAD-negative cells, determined by flow cytometry. Data are expressed as mean±s.e.m. * P <0.05 (Student’s t -test; n =3–4 independent experiments). Full size image Here, we show that loss of Pink1 reprograms glucose metabolism and this is likely to meet the bioenergetic requirements for the enhanced proliferation observed in Pink1 knockout proliferating cells such as fibroblasts. Moreover, we have also identified ROS-mediated HIF1α stabilization as the molecular mechanism responsible for this metabolic adaptation. According to our results obtained with mitochondrial-tagged antioxidant enzymes, mitochondrial-derived ROS are likely to play a key role in HIF1α stabilization. However, the involvement of cytosolic ROS in this effect cannot be discarded. In fact, decreased catalase and peroxiredoxin have been linked to the loss of PINK1 in other vertebrates such as zebrafish [18] . This may also account for the ROS increase observed by us in Pink1 -null cells. In addition, a decrease in Hif1 α mRNA has been previously reported in the Pink1 KO zebrafish [24] , and in Pink1 KO MEF and neurons on hypoxia [25] . Here, we detected higher HIF1α protein levels in spite of a lower Hif1 α mRNA abundance under normoxia that could represent a compensatory response to HIF1α stabilization. The upregulation of glucose metabolism on Pink1 loss reported here apparently contrasts with a previous study reporting impaired glucose uptake in Pink1 KO neurons [18] , [26] . While reasons for this discrepancy are unclear, it should be noted that we found both increased glucose uptake and glycolysis rates at ~5 mM glucose concentration, instead at the very low (0–2 mM) glucose concentrations previously used [18] , [26] . Furthermore, we confirmed the increased glucose consumption using in vivo settings, as well as the requirement for HIF1α-enhanced glycolysis to maintain the high proliferative status of Pink1 -null cells. We were surprised that the molecular mechanism identified in this study results in a proliferative phenotype in dividing Pink1 KO cells. Interestingly, PD patients harbouring mutant PINK1 were reported to have increased astroglial proliferation [27] , which could be accounted for by the metabolic alterations described here. In line with this observation, it has been shown that the loss of function of the downstream PINK1 target, PARKIN [5] , [6] —as well as the loss of function of other PD-linked genes—is associated with increased cancer prevalence [28] . Therefore, it seems likely that PINK1 regulates cell proliferation through PARKIN. In addition, our data, showing enhanced proliferating activity of neural stem cells in the Pink1 -null mice brains, suggests a potentially unexpected key regulatory role for PINK1 in the metabolic adaptation of stem cells. Whether PD-relevant loss-of-function mutations on the PINK1 gene confer the high glycolytic phenotype that we describe here deserves further investigation; however, this is likely to be the case since such mutations also lead to mitochondrial oxidative phosphorylation defects [12] that are responsible for the switch from mitochondrial oxidative to glycolytic metabolism [16] . Some PINK1 single nucleotide polymorphic genotypes are associated with type 2 diabetes and obesity [29] , thus further studies focusing on glucose homeostasis and PD may be worth pursuing. Besides contributing to the observed enhanced proliferative rates detected in Pink1-null fibroblasts, the metabolic reprogramming observed on loss of Pink1 could also sustain mitochondrial proliferation in non-dividing cells such as neurons. In line with this concept, pink1 mutant flies activate a signalling pathway that attempts to compensate for mitochondrial dysfunction by inducing mitochondrial proliferation in post-mitotic cells [30] . The metabolic re-wiring identified in our study may also contribute to cellular damage on PINK1 loss. In this context, post-mitotic neurons subjected to increased glycolytic rate show oxidative stress-mediated neurodegeneration as a consequence of a compensative decreased PPP rate [15] . Our data showing such a PPP to glycolysis shift in Pink1 -deficient cells, including neurons, support the notion that such a mechanism likely contributes to the Pink1 loss-associated neurodegeneration in PD. Ethical statement regarding the use of animals Mice were bred at the Animal Experimentation Unit of the University of Salamanca, and all protocols were approved by the Bioethics Committee of the University of Salamanca in accordance with the Spanish legislation (RD53/2013). Pink1 knockout mice were generated by Lexicon Genetics (The Woodlands, Texas, USA); back-crossed for at least nine generations with C57Bl/6J WT mice for the experiments and bred under homozygosis. Cell cultures MEF were prepared from fetal (E13.5) Pink1 −/− ( Pink1 KO) and Pink1 +/+ (WT) offspring. Cells were seeded (10 5 cells cm −2 ) in high glucose (25 mM) DMEM (Sigma, Madrid, Spain) with 10% fetal calf serum (Roche Diagnostics, Heidelberg, Germany) and L-glutamine (4 mM), and incubated at 37 °C in a humidified 5% CO 2 -containing atmosphere. Cortical neurons in primary culture were prepared from fetal (E15.5) WT and PINK1 KO mice. Cells were seeded at 1.8 × 10 5 cells cm −2 in cell culture plastic dishes previously coated with poly-D-lysine (15 μg ml −1 ) in neurobasal medium containing 2% of B-27 supplement (Gibco Brl-Life Technologies, Grand Island, NJ, USA) and 2 mM L-glutamine. Neurons were incubated at 37 °C in a humidified 5% CO 2 -containing atmosphere; at day second, the medium was replaced and neurons were used on the seventh or eighth day in vitro . RNA interference To knockdown HIF1α, we used the stealth/siRNA ( siHif1 α) duplex oligonucleotide 5′-CAAGCAGCAGGAAUUGGAACAUUAU-3′; as controls ( siControl ), we used the scrambled non-sense siRNA 5′-CAACGAGGAUAAGGUCAAUAGCUAU-3′ (Invitrogen, Paisley, UK). Plasmids To confine the expression of the antioxidant enzymes GCL and catalase to mitochondria, the mitochondrial-tagged full-length cDNA encoding GCL ( mitoGCL ), generated in our laboratory as described [23] , and that of catalase ( mitoCAT ), a generous gift from J. A. Enriquez (Centro Nacional de Investigaciones Cardiovasculares, Madrid, Spain, were used. Both mitoGCL and mitoCAT were subcloned into pIRES2–EGFP (Invitrogen) for transfections. As controls, we used the empty plasmid (pIRES2–EGFP). Full-length cDNA encoding human Hif1 α was a generous gift from S. Cadenas (Centro de Biología Molecular Severo Ochoa, Madrid, Spain). Site-directed mutagenesis A mutant form of Hif1 α cDNA refractory to siHif1 α was generated using the site-directed mutagenesis QuikChange XL kit (Stratagene, La Jolla, CA, USA), followed by Dpn I digestion. The forward and reverse oligonucleotides of the sequence 5′-TCACTTTTTCAAGC T GT T GG G AT C GG G AC T TTATTACAGCAGCC-3′, carrying silent third-codon base point mutations (mutant nucleotides underlined) was used. Cell transfections and treatments Transfection of MEF or neurons with siRNA duplexes were performed using Lipofectamine RNAiMAX reagent (Life Technologies), using 100 nM (final concentration) of the siRNA following the manufacturer’ instructions, and cells were used after 3 days. For plasmid transfections, 1.6 μg (per 10 3 cells) of the plasmid was mixed with 1 μM polyethylenimine (Sigma) and preincubated for 10 min at room temperature in Optimem medium (Invitrogen). Cells were then incubated with this polyethylenimine/DNA-containing mixture at 37 °C for 1 h, followed by washing with PBS and further incubated in the corresponding culture medium for 24 h. The full-length cDNA encoding human Hif1 α, or its siHif α-refractory mutant form (obtained by site-directed mutagenesis as described above), were also used in co-transfection using Lipofectamine RNAiMAX, each with siHif1 α or siControl for 24 h. In some experiments, MEF cells were incubated with GSH-E) (100 μM for 24 h) or with 2-deoxy-D-glucose (2DG) (1 mM for 72 h). Assessment of cell proliferation This was achieved by BrdU incorporation into DNA followed by flow cytometric analysis after a 3-h pulse with BrdU (10 mg ml −1 ) using the APC BrdU Flow Kit (Becton Dickinson Biosciences, Franklin Lakes, NJ, USA). The proportions of cell cycle phases were also determined by flow cytometric analyses of 7-amino-actinomycin D (7-AAD)-stained cells. Cell proliferation was also confirmed by direct counting under light microscopy. Real transcriptase quantitative PCR analysis This was performed in total RNA samples, purified from MEF or neurons using a commercially available kit (Sigma), utilizing the Power SYBR Green RNA-to-C T 1-Step kit (Applied Biosystems, Township, USA). Reverse transcription was performed for 30 min at 48 °C, and PCR conditions were 10 min at 95 °C followed by 40 cycles of 15 s at 95 °C plus 1 min at 60 °C using the primers previously described [31] ( Supplementary Table 2 ) (purchased from Thermo Scientific, Offenbach, Germany). The mRNA abundance of each transcript was normalized to the ß-actin mRNA abundance obtained in the same sample. The resulting normalized values of the Pink1 knockout samples were expressed as the fold change compared with the corresponding normalized values of the WT samples. MicroRNA array RNA was prepared from the cerebral cortex of 6-month-old male mice (eight samples in total, four replicates for each genotype). The RNA quality was confirmed using an Agilent 2100 Bioanalyzer. Detailed experimental protocols and raw data were deposited in ArrayExpress under accession E-MTAB-2462 . Differential expression was analysed using R/Bioconductor through standard analysis pipelines. Western blot Cells or muscle tissue were lysed in 2% sodium dodecyl sulphate, 2 mM EDTA, 2 mM EGTA, 50 mM Tris, pH 7.5, supplemented with phosphatase inhibitors (1 mM Na 3 VO 4 , 50 mM NaF) and protease inhibitors (100 μM phenylmethylsulphonyl fluoride, 50 μg ml −1 anti-papain, 50 μg ml −1 pepstatin, 50 μg ml −1 amastatin, 50 μg ml −1 leupeptin, 50 μg ml −1 bestatin and 50 μg ml −1 soybean trypsin inhibitor), stored on ice for 30 min and boiled for 10 min. Aliquots of the extracts were subjected to sodium dodecyl sulphate polyacrylamide gel electrophoresis (MiniProtean, Bio-Rad, Hercules, CA, USA) and blotted with antibodies overnight at 4 °C. Signal detection was performed with an enhanced chemiluminescence kit (ECL Plus western blotting detection reagent from GE Healthcare, Piscataway Township, NJ, USA). Antibodies used were anti-HIF1α (1:250; ab16066; Abcam, Cambridge Science Park, Cambridge, UK), anti-PINK1 (1:500; BC100-494; Novus Biologicals, Littleton, CO, USA), anti-HK2 (1:500; sc-6521; Santa Cruz Biotechnology, Dallas, TX, USA), anti-β-actin (1:30,000; A5441; Sigma), α-tubulin (1:2,000; T5168, Sigma), anti-GAPDH (1:40,000; AM4300; Life Technologies, Grand Island, NY, USA), anti-PDK1 (1:1,000; ADI-KAP-PK112; Stressgen-Enzo Life Sciences, Farmingdale, NY, USA), anti-GLUT1 (1:500; 07-1401; EMD Millipore Corporation, Billerica, MA, USA) and anti-GLUT3 (1:250; sc-74497; Santa Cruz Biotechnologies). After incubation with horseradish peroxidase-conjugated goat anti-rabbit IgG (Santa Cruz Biotechnologies), goat anti-mouse IgG (Santa Cruz Biotechnologies), or rabbit anti-goat IgG (Santa Cruz Biotechnologies) (all at 1:10,000 dilution), membranes were immediately incubated with the enhanced chemiluminescence kit SuperSignal West Dura (Pierce, Thermo Scientific, Illinois, USA) for 5 min or Immobilon Western Chemiluminescent HRP Substrate (Merck Millipore; Darmstadt, Germany) for 1 min, before exposure to Kodak XAR-5 film for 1–5 min, and the autoradiograms scanned. Biologically independent replicates (2–5) were always performed; a representative western blot is shown in the main article, and the replicates are shown in the Supplementary Information . The protein abundances were measured by densitometry of the bands on the films using ImageJ 1.48u4 software (National Institutes of Health, USA), and were normalized against the corresponding loading control (ß-actin or α-tubulin). The protein abundance was calculated as the ratio of the normalized protein of the Pink1 KO cells relative to that of the WT, and the resulting values were used for the statistical analysis. Mitochondrial function parameters and ROS determination Cells were collected and suspended in 0.1 M potassium phosphate buffer (pH 7.0). After freeze/thawing three times to ensure cellular disruption, NADH-CoQ1 reductase (complex I), succinate-cytochrome c reductase (complex II–III), cytochrome c oxidase (complex IV) and citrate synthase activities were determined as previously described [32] PDH activity was determined in intact mitochondria, isolated as previously described [23] as the rate of [1- 14 C]pyruvate decarboxylation to 14 CO 2 (ref. 33 ). The mitochondrial membrane potential (Δψ m ) was assessed using MitoProbe DiIC 1 (5) Assay Kit for flow cytometry (Molecular Probes Europe BV, Leiden, Netherlands). Δψ m values were expressed as percentages, using carbonyl cyanide 4-(trifluoromethoxy)phenylhydrazone (FCCP; 10 μM) to define the 0% Δψ m values. Mitochondrial superoxide was assessed in intact cells using the fluorescent MitoSox probe (Invitrogen) by flow cytometry, and whole cell-derived H 2 O 2 was measured, in intact cells, using the fluorescent AmplexRed probe (Invitrogen), following the manufacturers’ instructions. Rate of glucose uptake Cultured cells were washed twice with PBS and incubated in a Krebs-Ringer phosphate glucose (KRPG) buffer (145 mM NaCl, 5.7 mM Na 2 PO 4 , 4.86 mM KCl, 0.54 mM CaCl 2 , 1.22 mM MgSO 4 and 5.0 mM glucose, pH 7.4) at 37 °C in the CO 2 incubator. After 1 h, 10 μl of [1- 14 C]-2-deoxyglucose (60 mCi mmol −1 ; Amersham) was added to the KRPG buffer to a final radioactivity of 0.2 μCi ml −1 and cells were incubated for a further 5, 15 and 25 min. At the end of each of these periods of time, the radioactive media was removed and subsequently used to assess the specific radioactivity; cells were rapidly washed three times with ice-cold PBS and immediately lysed with 0.6 ml of 0.1 M NaOH. A 0.5 ml lysate aliquot was used for radioactivity determination using a liquid scintillation counter, and the rest was used to determine protein concentration. The rate of glucose uptake was calculated from the radioactivity versus time regression slopes, which were linear up to the 25 min of incubation. At least four different wells were used for each sample, and at least three different culture preparations were used per condition. Rates of glycolysis and PPP These were measured in suspended cells (4–5 × 10 5 cells), incubated in KRPG buffer in the presence of 5 μCi of D-[3- 3 H]glucose, 0.5 μCi ml −1 of D-[1- 14 C]glucose or 1 μCi ml −1 of [6- 14 C]glucose and 5 mM D-glucose in sealed vials. The glycolytic flux was measured by assaying the rate of 3 H 2 O production from [3- 3 H]glucose, and the PPP flux as the difference between [1- 14 C]glucose and [6- 14 C]glucose incorporated into 14 CO 2 , as detailed previously [15] . In vivo blood lactate production was determined 15 min after a tail vein injection of 5 μCi of [U- 14 C]glucose. Blood [U- 14 C]lactate was separated from [U- 14 C]glucose by ion exchange chromatography (Dowex AG-1 × 8) as we previously described [15] , and measured by liquid scintillation counting. Lactate and glucose concentrations were measured in either cell culture media at the indicated times, or in deproteinized blood samples, by enzymatic analysis spectrophotometrycally [15] . Flow cytometric analysis of apoptotic neuronal death Neurons were carefully detached from the plates using 1 mM EDTA (tetrasodium salt) in PBS. APC-conjugated annexin-V and 7-amino-actinomycin D (7-AAD) (Becton Dickinson Biosciences) were used to determine quantitatively the percentage of apoptotic neurons by flow cytometry. Cells were stained with annexin V-APC and 7-AAD in binding buffer (100 mM HEPES, 140 mM NaCl, 2.5 mM CaCl 2 ), according to the manufacturer's instructions, and 3 × 10 5 cells were analysed, in four replicates per condition, on a FACScalibur flow cytometer (15 mW argon ion laser tuned at 488 nm; CellQuest software, Becton Dickinson Biosciences). The annexin V-APC-stained neurons that were 7-AAD-negative were considered to be apoptotic. The analyser threshold was adjusted on the flow cytometer channel to exclude most of the subcellular debris to reduce the background noise owing to the neurite disruption during neuronal detaching. Data were expressed as percentages. Inmunohistochemistry After deep anaesthesia, mice were perfused intraaortically with 0.9% NaCl, followed by 4% (w/v) paraformaldehyde, 0.2% (w/v) picric acid in 0.1 M phosphate buffer (pH 7.4). Brains were dissected and post fixed overnight and cryoprotected before 20-μm thick coronal sections were obtained with a freezing-sliding cryostate (Leica CM 1950 AgProtect, Leica, Nussloch, Germany). Sections were incubated with anti-Sox2 antibody (1:4,000; Abcam, ab79351) that stains stem cells, overnight at 4 °C, followed by anti-Ki67 antibody (1:200; Clone SP6; Thermo Scientific), which is expressed in proliferating cells, for 1 h at room temperature. Sections were further incubated with Cy3 anti-rabbit for Sox, and Cy2 anti-mouse for Ki67, followed by DAPI staining. Mounted sections were examined by epifluorescence under a Nikon Inverted microscope (Eclipse Ti-E, Japan) equipped with a precentered fibre illuminator (Nikon Intensilight C-HGFI, Tokyo, Japan) and B/W CCD digital camera (Hamamatsu ORCA-ER, Hamamatsu, Japan). The total number of cells (DAPI + ) and Ki67 + /Sox2 + cells were counted in 0.3 mm 2 sections from three slices/mouse. Protein determinations Protein concentrations were determined in the cell suspensions, lysates or in parallel cell culture incubations after solubilization with 0.1 M NaOH. Protein concentrations were determined as described [34] using bovine serum albumin as standard. Statistical analysis All measurements in cell culture were carried out at least in three different culture preparations, and the results are expressed as the mean±s.e.m. For in vivo experiments, we used at least four animals per condition. For the comparisons between two groups of values, the statistical analysis of the results was performed by the Student’s t -test. For multiple values comparisons, we used one-way analysis of variance followed by Bonferroni test. The statistical analysis was performed using the SPSS 16.0 software for Macintosh. In all cases, P <0.05 was considered significant. Accession codes : Microarray raw data are available in the ArrayExpress database ( www.ebi.ac.uk/arrayexpress ) under the accession number E-MTAB-2462 . How to cite this article : Requejo-Aguilar, R. et al. PINK1 deficiency sustains cell proliferation by reprogramming glucose metabolism through HIF1. Nat. Commun. 5:4514 doi: 10.1038/ncomms5514 (2014).